Structures of an intramembrane vitamin K epoxide reductase homolog reveal control mechanisms for electron transfer The intramembrane vitamin K epoxide reductase (VKOR) supports blood coagulation in humans and is the target of the anticoagulant warfarin. VKOR and its homologues generate disulphide bonds in organisms ranging from bacteria to humans. Here, to better understand the mechanism of VKOR catalysis, we report two crystal structures of a bacterial VKOR captured in different reaction states. These structures reveal a short helix at the hydrophobic active site of VKOR that alters between wound and unwound conformations. Motions of this ‘horizontal helix’ promote electron transfer by regulating the positions of two cysteines in an adjacent loop. Winding of the helix separates these ‘loop cysteines’ to prevent backward electron flow. Despite these motions, hydrophobicity at the active site is maintained to facilitate VKOR catalysis. Biochemical experiments suggest that several warfarin-resistant mutations act by changing the conformation of the horizontal helix. Taken together, these studies provide a comprehensive understanding of VKOR function. Human vitamin K epoxide reductase (VKOR) is an integral membrane protein that supports the activity of vitamin K-dependent proteins, which are involved in a variety of physiological processes including blood coagulation, bone mineralization [1] , energy metabolism [2] , calcium homeostasis, signal transduction, cell growth and apoptosis [3] , [4] . VKOR is the target of warfarin, the most commonly used anticoagulant that treats and prevents deep vein thrombosis, pulmonary embolism, stroke and myocardial infarction. VKOR functions through the vitamin K cycle in the endoplasmic reticulum (ER). The cycle begins with the γ-carboxylation of several glutamic acids in vitamin K-dependent proteins such as coagulation factors; this post-translational modification is required for their activation at the sites of injury [5] . The γ-carboxylase activity results in the epoxidation of the vitamin K hydroquinone. The role of VKOR is to regenerate the hydroquinone by reducing the vitamin K epoxide, with a vitamin K quinone serving as an intermediate. Each step of the reduction results in the formation of a disulphide bond at the active site of VKOR. To regenerate the reduced active site, VKOR requires partner proteins that pass the disulphide to newly synthesized proteins containing free cysteines [6] , [7] . Homologues of VKOR have been found in bacteria, archaea, plants, insects and mammals [8] . Bacterial VKOR homologues constitute a large family of enzymes that generate disulphide bonds in the periplasmic space, a function similar to that of a DsbB protein [9] . Archaeal VKORs promote disulphide-bond formation in cytoplasmic proteins to improve their stability at extreme conditions [10] . In Arabidopsis , a VKOR homologue likely catalyses disulphide-bond formation in the thylakoid [11] . A recent study found that VKOR also contributes to disulphide-bond formation in the ER lumen of mammals [12] . Knockdown of VKOR expression in combination with other ER-associated disulphide-bond-forming enzymes results in complete cell death. Taken together, it becomes increasingly clear that VKOR is broadly involved in disulphide-bond formation, which is crucial for the maturation of many secretory proteins by ensuring their timely folding and by preventing protein aggregation [13] . We previously determined the 3.6-Å crystal structure of a bacterial VKOR homologue from Synechococcus sp. (ssVKOR) with its autologous reducing partner, a thioredoxin-like (Trx) domain [14] . At the VKOR active site, a CXXC motif (Cys130 and Cys133) is in close proximity to a quinone molecule. Another pair of conserved cysteines (Cys50 and Cys56) is located in a loop region, which is followed by a short helix we termed the horizontal helix ( Fig. 1a ). These ‘loop cysteines’ were proven to be essential in mediating disulphide exchange between the active sites of ssVKOR and Trx [14] , which contains another CXXC motif (Cys209 and Cys212). The disulphide exchange is accompanied by the sequential transfer of electrons from Trx to the VKOR domain ( Fig. 1a ). The electron-transfer intermediates can be captured by mutating one cysteine in a pair to generate a free thiol, which can subsequently reduce its target disulphide ( Fig. 1b ). Using this strategy, we determined this previous structure with a Cys56Ala mutation captured in a state where electrons are being transferred from the Trx domain to the loop cysteines. 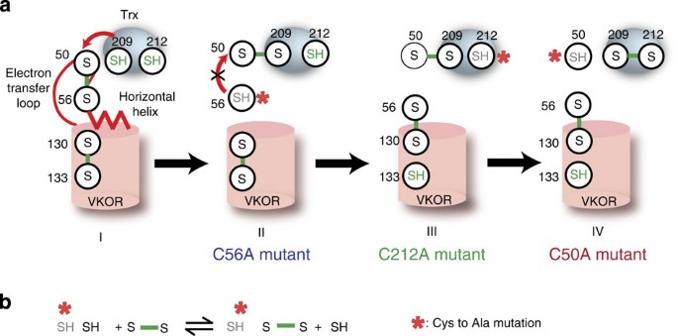Figure 1: The electron transfer pathway. The electron transfer process can be followed by the changes of sulfhydryls (coloured in green). (a)State I:at this initial state, Cys209 and Cys212 at the active site of the Trx domain have been reduced by nascent proteins. The Cys209 and Cys212 sulfhydryls will subsequently reduce the Cys50-Cys56 disulphide.State II:Cys209/Cys212 forms a mixed disulphide with Cys50/Cys56. The red arrow shows a possible backward reaction in which the Cys56 attacks the Cys50-Cys209 disulphide. A Cys56Ala mutation (red asterisk) directly prevents this backward attack (black cross) and stabilizes the Cys50-Cys209 disulphide.State III:physical separation of Cys56 from Cys50-Cys209 disulphide may also prevent the backward attack. The free Cys56 can interact with Cys130/Cys133 at the active site of VKOR, leaving behind the Cys50/Cys209/Cys212. A Cys212Ala mutation (red asterisk) can stabilize this state.State IV:the free Cys50 reduces the Cys56-Cys130 disulphide. A Cys50Ala mutation prevents this attack and stabilizes the Cys56-Cys130 disulphide. (b) The strategy of capturing electron-transfer intermediates. A single mutation (red asterisk) in a cysteine pair will generate a free thiol in the other cysteine, which subsequently reduces another cysteine pair and forms an alternative disulphide. Figure 1: The electron transfer pathway. The electron transfer process can be followed by the changes of sulfhydryls (coloured in green). ( a ) State I: at this initial state, Cys209 and Cys212 at the active site of the Trx domain have been reduced by nascent proteins. The Cys209 and Cys212 sulfhydryls will subsequently reduce the Cys50-Cys56 disulphide. State II: Cys209/Cys212 forms a mixed disulphide with Cys50/Cys56. The red arrow shows a possible backward reaction in which the Cys56 attacks the Cys50-Cys209 disulphide. A Cys56Ala mutation (red asterisk) directly prevents this backward attack (black cross) and stabilizes the Cys50-Cys209 disulphide. State III: physical separation of Cys56 from Cys50-Cys209 disulphide may also prevent the backward attack. The free Cys56 can interact with Cys130/Cys133 at the active site of VKOR, leaving behind the Cys50/Cys209/Cys212. A Cys212Ala mutation (red asterisk) can stabilize this state. State IV: the free Cys50 reduces the Cys56-Cys130 disulphide. A Cys50Ala mutation prevents this attack and stabilizes the Cys56-Cys130 disulphide. ( b ) The strategy of capturing electron-transfer intermediates. A single mutation (red asterisk) in a cysteine pair will generate a free thiol in the other cysteine, which subsequently reduces another cysteine pair and forms an alternative disulphide. Full size image Despite VKOR’s widespread role in assisting oxidative protein folding and blood coagulation, the physical mechanisms of electron transfer in VKOR remain unclear. The loop cysteines (Cys50/Cys56) have to change conformation in order to gain access to the two active sites of the VKOR and Trx domains, which are separated by a 16-Å distance. In addition, how VKOR promotes an electron flow in the forward direction [15] , [16] is completely unknown. Elucidating these mechanisms requires structures to be determined of other VKOR electron-transfer states, especially the state when the electrons are transferred from the loop cysteines to the active site of VKOR. Here we report two new structures of ssVKOR captured in different conformational states to visualize later stages of the electron-transfer pathway. Comparison of the structural intermediates reveals the importance of the horizontal helix that undergoes unwinding motions to promote electron transfer. The N -terminal part of this helix acts like a spring: its unwound state facilitates the electron transfer from the Trx active site, and its helical state allows the electron transfer to the VKOR active site. Winding of the helix also separates the loop cysteines to prevent futile electron transfer in the reverse direction. During these motions, the hydrophobic residues of the horizontal helix remain covering the quinone-binding pocket and maintain a low-dielectric environment that is likely important for quinone reduction and disulphide-bond formation in VKOR. Biochemical experiments support this spring model and reveal that several warfarin resistance mutations may act by altering the orientation of the horizontal helix. Structure determination We made two constructs that would likely capture later stages of the electron transfer ( Fig. 1a ): a Cys50Ala mutant containing a Cys56 thiol, which may reduce Cys130-Cys133 at the active site of ssVKOR (state IV), and a Cys212Ala mutant containing a Cys209 thiol, which may reduce Cys50-Cys56 in the loop region. If the electron transfer continues, the reduced Cys56 thiol will subsequently react with the Cys130-Cys133 disulphide (state III). The Cys50Ala crystals diffracted to 2.8 Å ( Supplementary Fig. 1 ) after dehydration, and the molecular replacement (MR) solution was found by using individual domains from the Cys56Ala structure [14] as search models. Omit maps with a series of deletions (see Methods ) were used for manual building of the Cys50Ala model ( Fig. 2 ), which was refined to an R free value of 24.5% ( Table 1 ). An omit map, calculated with the deletion of the loop/helix region connecting TM1 and TM2 from the MR model, generated electron density indicating a conformational change in this region ( Fig. 3 ). 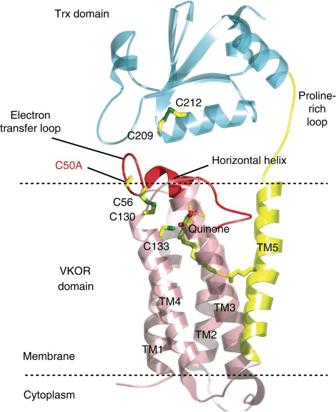Figure 2: Overall structure of the ssVKOR in state IV. The transmembane helices (TM1–4) homologous to the mammalian VKOR are coloured in pink, the Trx domain in blue and the electron-transfer loop and the horizontal helix in red. The dotted lines indicate the membrane boundary. The quinone and conserved cysteines are labelled. Figure 2: Overall structure of the ssVKOR in state IV. The transmembane helices (TM1–4) homologous to the mammalian VKOR are coloured in pink, the Trx domain in blue and the electron-transfer loop and the horizontal helix in red. The dotted lines indicate the membrane boundary. The quinone and conserved cysteines are labelled. Full size image Table 1 Data collection, phasing and refinement statistics*. 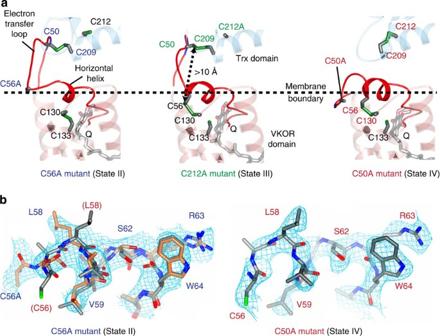Figure 3: Conformational changes in the loop/helix region between different electron transfer states. (a) Zoomed views of the Cys56Ala (left), Cys212Ala (middle) and Cys50Ala (right) structures. Conformational changes are observed in the electron-transfer loop and horizontal helix. (b) Left, electron density map (contoured at 1σ) of Cys56Ala horizontal helix. The Cys56Ala structure (gold) is superimposed with Cys50Ala structure (grey). The difference becomes evident towards theN-terminus of the horizontal helix: from Leu58 to Cys56 (residues of the Cys50Ala construct labelled in parenthesis). Right, electron density map (contoured at 1σ) of Cys50Ala horizontal helix (grey). Full size table Figure 3: Conformational changes in the loop/helix region between different electron transfer states. ( a ) Zoomed views of the Cys56Ala (left), Cys212Ala (middle) and Cys50Ala (right) structures. Conformational changes are observed in the electron-transfer loop and horizontal helix. ( b ) Left, electron density map (contoured at 1σ) of Cys56Ala horizontal helix. The Cys56Ala structure (gold) is superimposed with Cys50Ala structure (grey). The difference becomes evident towards the N -terminus of the horizontal helix: from Leu58 to Cys56 (residues of the Cys50Ala construct labelled in parenthesis). Right, electron density map (contoured at 1σ) of Cys50Ala horizontal helix (grey). Full size image The Cys212Ala mutant was crystallized, in a different space group, using high concentrations of lipid and detergent [17] . These crystals diffracted only to 4.2 Å. Although the resolution is low, an omit map showed the regeneration of the entire loop region ( Supplementary Fig. 2 ) and we were able to roughly build the Cα trace of this loop ( Fig. 3a ). Owing to its higher accuracy, the refined 2.8-Å structure was used to re-calculate omit maps for the Cys56Ala mutant; these model maps were very similar to the experimental map previously obtained [14] . Thus, the electron density at the horizontal helix ( Fig. 3b ) of the Cys56Ala mutant was confirmed by two independent phasing methods. In sum, three electron-transfer states have been captured, in which the structures of Cys56Ala, Cys212Ala and Cys50Ala mutants ( Fig. 3a ) represent the states II, III and IV ( Fig. 1a ), respectively. Overall structures The Cys50Ala structure ( Fig. 2 ) represents the state in which electrons are transferred from Cys56 to the VKOR active site. Compared with the Cys56Ala structure in state II, the Trx domain has rotated by 20 degrees towards the VKOR domain. This rigid body rotation is hinged through a proline-rich region that connects the two domains. Rotation of the Trx domain is probably induced by a downward flipping of the electron-transfer loop (containing Cys50/Cys56), which would otherwise prevent the movement of the Trx domain. The Cys212Ala structure ( Fig. 3a , middle), in state III, has some characteristics from both the Cys56Ala (state II) and Cys50Ala (state IV) structures. The electron-transfer loop has its N -terminal part inserted into the Trx-binding groove and its C -terminal part is close to the VKOR active site. Importantly, Cys50 and Cys56 are now separated by a distance of >10 Å after the Cys50-Cys56 disulphide is reduced by the free Cys209. This physical separation may prevent backward electron transfer. In these different electron-transfer states, the VKOR and Trx domains retain their architectures, a 4-helix bundle and a thioredoxin fold, respectively ( Fig. 2 ). However, conformational changes are observed in the electron-transfer loop and in the horizontal helix that covers on top of the VKOR active site ( Fig. 3 ). Conformational changes in different electron transfer states The electron-transfer loop undergoes a large conformational change between different states. In the Cys56Ala and Cys212Ala structures ( Fig. 3a ), the N-terminal part of the loop binds to a small binding groove of the Trx domain through hydrophobic interactions and a disulphide bond of Cys50-Cys209. In contrast, this entire loop in the Cys50Ala structure flips down using Glu44 as a hinge; Glu44 is at the C -terminal end of the TM1 helical region. Residues Ala47 to Phe49 may have inserted into the membrane phase, as judged by their positions relative to the TM region. Conformational changes in the horizontal helix are clear in the two structures of higher resolution ( Fig. 3b ). In the Cys50Ala structure, the N -terminal end of the horizontal helix becomes more compact when Cys56 and Cys130 form a disulphide bond. The horizontal helix adopts a typical α-helical conformation, and four hydrogen bonds could be formed from Gly55 to Ser62. In contrast, in the Cys56Ala structure, the horizontal helical region adopts an unwound conformation; the Cα trace is no longer α-helical and only two hydrogen bonds are potentially formed. When these two structures are superimposed at the horizontal helix region, the C-terminal residues, Ser62 to Trp64, superimposes relatively well; however, the difference becomes obvious from Leu58 towards N-terminus of the horizontal helix ( Fig. 3b , left). The conformational changes of the horizontal helix in different states suggest that VKOR uses this helix to promote electron transfer. Coordination of the horizontal helix and the loop cysteines How does the winding and unwinding motions of the horizontal helix promote electron transfer? Since Cys56 is located at the exact N-terminal end of this helix, we postulated that the motions of horizontal helix may drag Cys56 back and forth for electron transfer. To illustrate this mechanism, we made a series of constructs that inserted residues between Cys56 and the horizontal helix. The rate of electron transfer was determined by using reduced and unfolded RNaseA as the electron donor [14] . The RNaseA reduces the Trx active site, and the loop cysteines subsequently transfer the electrons to the VKOR active site. In contrast, the electron transfer can be bypassed by using dithiothreitol (DTT) as the reductant, which is membrane-permeable and can directly reduce the VKOR active site. Using this assay, we found that all of the insertion mutations significantly lowered the rate of electron transfer; however, the rate of vitamin K reduction at the active site was largely unaffected ( Fig. 4 ). A control experiment using Cys56Ala blocked the vitamin K reduction promoted by RNaseA, but not by DTT. 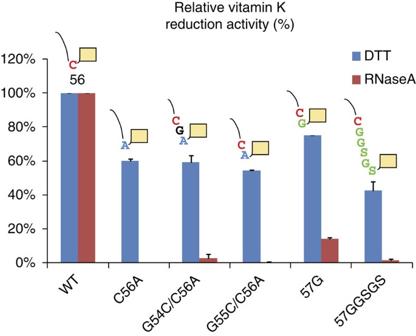Figure 4: Proximity of Cys56 and horizontal helix is required for electron transfer. Inserting residues between Cys56 and the horizontal helix lowers the rate of electron transfer, which is initiated by RNaseA reduction of the Trx domain (red bars). The DTT reduction at the active site (blue bars) is largely unchanged. Error bars represent s.e. of three duplicated measurements. Mutants with insertion between Cys56 and the horizontal helix (orange box) were made by either moving Cys56 (red) to a different position on the polypeptide chain through mutations (Gly55Cys/Cys56Ala, Gly54Cys/Cys56Ala) or by inserting a flexible linker (Gly or Gly-Gly-Ser-Gly-Ser) between Cys56 and Gly57. The mutated residues are shown in blue and the inserted residues in green. Figure 4: Proximity of Cys56 and horizontal helix is required for electron transfer. Inserting residues between Cys56 and the horizontal helix lowers the rate of electron transfer, which is initiated by RNaseA reduction of the Trx domain (red bars). The DTT reduction at the active site (blue bars) is largely unchanged. Error bars represent s.e. of three duplicated measurements. Mutants with insertion between Cys56 and the horizontal helix (orange box) were made by either moving Cys56 (red) to a different position on the polypeptide chain through mutations (Gly55Cys/Cys56Ala, Gly54Cys/Cys56Ala) or by inserting a flexible linker (Gly or Gly-Gly-Ser-Gly-Ser) between Cys56 and Gly57. The mutated residues are shown in blue and the inserted residues in green. Full size image The horizontal helix and warfarin-resistant mutations As the horizontal helix is important for tethering Cys56 to the membrane, we examined the extent to which the helix is buried inside the membrane. We used a labelling method developed for DsbD and DsbB [18] , [19] : a residue mutated to cysteine is first modified by a membrane-impermeable maleimide probe, AMS (4-acetamido-4′-maleimidylstilbene-2,2′-disulfonic acid; 0.54 kDa). The protein is subsequently denatured, and unblocked cysteines are labelled by a larger maleimide probe, MalPEG 5 kDa. Thus, the relative extent of modification by AMS and MalPEG shows the membrane accessibility of the mutated residue. Using this method, we found AMS was capable of labelling residues Asp57Cys, Leu58Cys, Ser61Cys and Ser62Cys located on the aqueous side of the horizontal helix ( Fig. 5a ). However, the residues Val59Cys and Leu60Cys located on the membrane side were not efficiently labelled. Therefore, it seems that the horizontal helix is partially buried in the membrane. 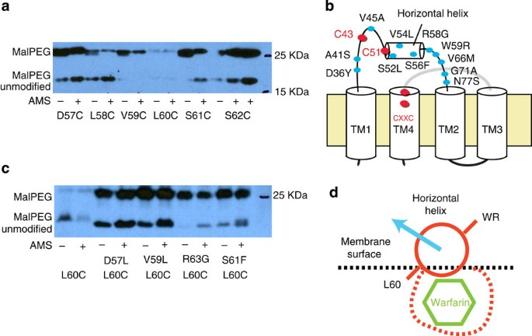Figure 5: Membrane accessibility of the horizontal helix and effect of warfarin-resistant mutations (WRs). (a) Residues on the horizontal helix show different accessibilities to AMS, a membrane-impermeable probe. (b) Many WRs (blue circles) are located between TM1 and TM2 in human VKOR. (c) Corresponding WRs in ssVKOR changing the AMS labelling of Leu60Cys. The mutant proteins are initially labelled by membrane-impermeable AMS (0.5 kDa). After TCA precipitation, the unblocked cysteine is modified by MalPEG (5 KDa). Thus, the relative extent of AMS and MalPEG labelling indicates the membrane accessibility of Leu60Cys. (d) These WRs may induce a movement of the flexible horizontal helix, which may cause resistance by altering the putative warfarin-binding pocket. Figure 5: Membrane accessibility of the horizontal helix and effect of warfarin-resistant mutations (WRs). ( a ) Residues on the horizontal helix show different accessibilities to AMS, a membrane-impermeable probe. ( b ) Many WRs (blue circles) are located between TM1 and TM2 in human VKOR. ( c ) Corresponding WRs in ssVKOR changing the AMS labelling of Leu60Cys. The mutant proteins are initially labelled by membrane-impermeable AMS (0.5 kDa). After TCA precipitation, the unblocked cysteine is modified by MalPEG (5 KDa). Thus, the relative extent of AMS and MalPEG labelling indicates the membrane accessibility of Leu60Cys. ( d ) These WRs may induce a movement of the flexible horizontal helix, which may cause resistance by altering the putative warfarin-binding pocket. Full size image Interestingly, several warfarin-resistant mutations identified in human and rodents have been mapped on or close to the horizontal helix of ssVKOR ( Fig. 5b ); patients having these resistant mutations show a significantly higher requirement for warfarin dosage [20] , [21] , [22] . Do these mutations affect the conformation of the horizontal helix? Using the method described above, we found that the Asp57Leu, Val59Leu, Ser61Phe and Arg63Gly in ssVKOR (corresponding to Ser52Leu, Val54Leu, Ser56Phe and Arg58Gly in human VKOR) all increased the membrane accessibility of Leu60Cys on the horizontal helix ( Fig. 5c ). The change of AMS modification to Leu60Cys can be explained by a movement of the horizontal helix that weakens its membrane association ( Fig. 5d ). In other words, the warfarin-resistant mutations appear to induce a conformational change in the horizontal helix region. VKOR active site The Cys50Ala structure at 2.8 Å resolution provides mechanistic insights into the quinone reduction and disulphide-bond formation at the VKOR active site. We observed continuous electron density connecting the quinone, VKOR’s CXXC motif and a loop cysteine ( Fig. 6a ). The densities show the disulphide-bonded forms of Cys56-Cys130 and Cys130-Cys133, and a covalent link between Cys133 and the quinone. The continuous density probably reflects an averaging effect because different molecules in the crystal can have alternative ways of forming a covalent bond. The orientation of the quinone is well defined by the density map, and in one alternative state Cys133 may link covalently to the C1 atom of the quinone ring ( Fig. 6b ). The C1 atom and the three sulphurs in Cys56, Cys130 and Cys133 are aligned in a straight line ( Fig. 6a ), a preferred orientation for the nucleophilic attack by a thiolate group [23] . The Met118 residue stacks at the bottom of the quinone ring and assists to position the quinone to react with Cys133 ( Fig. 6c ). Ser62, a residue conserved among all VKORs, is close to the quinone ring. Interestingly, Cys133 is buried in a hydrophobic pocket, which is formed by Val59 and Leu60 from the horizontal helix and Leu37, Met122 and Tyr132 from the transmembrane helices ( Fig. 6c ). 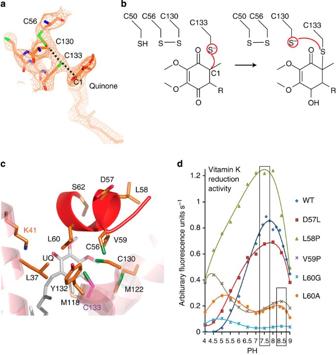Figure 6: The hydrophobic active site of VKOR. (a) Continuous electron density at the active site. The omit map (contoured at 1σ) is calculated using a partial model in which the quinone and all residues surrounding the active site are deleted. The regenerated electron density connects Cys56 in the electron-transfer loop, Cys130 and Cys133 at the active site, and the quinone. Alternative ways of covalent-bond formation are indicated by dashed lines. (b) The proposed chemistry for disulphide-bond formation. Left, the deprotonated Cys133 tholate attacks the C1 atom of the quinone. Right, Cys133 forms a covalently linked intermediate with the quinone, and the deprotonated Cys130 attacks this intermediate to form a disulphide bond. (c) Structure of the active site showing that Cys133 is surrounded by hydrophobic residues. (d) The DTT-driven vitamin-K reduction activity and pH optimum of ssVKOR mutants. Shifted pH optima are observed for Val59 and Leu60 mutant proteins, which are hydrophobic residues surrounding Cys133. However, this effect is not seen for mutations of nearby residues, Asp57 and Leu58. Figure 6: The hydrophobic active site of VKOR. ( a ) Continuous electron density at the active site. The omit map (contoured at 1σ) is calculated using a partial model in which the quinone and all residues surrounding the active site are deleted. The regenerated electron density connects Cys56 in the electron-transfer loop, Cys130 and Cys133 at the active site, and the quinone. Alternative ways of covalent-bond formation are indicated by dashed lines. ( b ) The proposed chemistry for disulphide-bond formation. Left, the deprotonated Cys133 tholate attacks the C1 atom of the quinone. Right, Cys133 forms a covalently linked intermediate with the quinone, and the deprotonated Cys130 attacks this intermediate to form a disulphide bond. ( c ) Structure of the active site showing that Cys133 is surrounded by hydrophobic residues. ( d ) The DTT-driven vitamin-K reduction activity and pH optimum of ssVKOR mutants. Shifted pH optima are observed for Val59 and Leu60 mutant proteins, which are hydrophobic residues surrounding Cys133. However, this effect is not seen for mutations of nearby residues, Asp57 and Leu58. Full size image VKOR activity and the hydrophobic pocket Since another disulphide-forming enzyme, DsbB, uses an essential arginine to assist catalysis by stabilizing the transition state ( Supplementary Fig. 4c ), we first investigated the role of basic residues in ssVKOR. Lys41 is not conserved among VKORs but is the only basic residue close (~4.5 Å) to the quinone ( Fig. 6c ). We found that the Lys41 mutants (Ser/Ala/Glu) of ssVKOR did not result in loss of much activity ( Supplementary Fig. 3 ). If a basic residue is not absolutely required, could the hydrophobic pocket in ssVKOR play a role in catalysis by activating the Cys133 thiol? Despite the conformational changes in different structures ( Fig. 3a ), the catalytic residue Cys133 (which interacts with the quinone) remains in the hydrophobic pocket. To test the importance of this hydrophobic environment, we exposed the Cys133 to water by shortening the side chains of residues (for example, mutate Leu60 to Ala) on the horizontal helix, which forms part of the hydrophobic pocket. Interestingly, not only did these mutants show a significant loss of activity, but the pH optimum of ssVKOR activity was also shifted from 7.5 to 8.5 ( Fig. 6d ). However, mutating the nearby residues, Asp57 and Leu58, which are not part of the hydrophobic pocket, did not have the same effect on the enzymatic activity. The Cys50Ala structure of ssVKOR at 2.8 Å resolution allowed a detailed analysis of an intramembrane enzyme that generates disulphide bonds. In the active site, a continuous electron density connects the thiol group of Cys133 with the C1 atom of the quinone ring ( Fig. 6a ), clearly demonstrating the proposed chemistry of the disulphide bond generation in VKOR [24] , [25] or DsbB [26] . In these models, a deprotonated thiolate serves as a nucleophile to attack the C1 group of the quinone, and rearrangement of the covalent bonds generates a disulphide ( Fig. 6b ). Compared with DsbB, ssVKOR probably uses a different mechanism to activate this catalytic thiol. DsbB has a hydrophilic pocket and uses an essential arginine to neutralize the negative charge of a deprotonated thiolate ( Supplementary Fig. 4c ), thereby stabilizing the transition state of the reaction [27] . In the ssVKOR structure, Lys41 is the only basic residue that is close to the active site but is not essential for activity ( Supplementary Fig. 3 ). Since thiol deprotonation correlates with its pKa, which is known to be very sensitive to the local environment [28] , [29] , the hydrophobic pocket in ssVKOR ( Fig. 6c ) may play a role in lowering the pKa of Cys133 for its deprotonation at neutral pH. A lowered thiol pKa in a hydrophobic environment has been suggested on the basis of theoretical calculations of thiol reactions [30] and has been observed in other membrane proteins [31] . When hydrophobic residues Val59 and Leu60 covering the active site are mutated and Cys133 is exposed to water, ssVKOR exhibits much lower enzymatic activity ( Fig. 6d ). The pH optimum in these mutants is shifted back to about 8.5, possibly reflecting a change in the thiol pKa, which is typically 8.7 in water but can be dramatically lowered in the microenvironment of a protein [32] . The hydrophobicity surrounding the catalytic cysteine is well conserved among VKOR homologues, suggesting a general mechanism to promote efficient catalysis in all VKORs. Deprotonation of this cysteine is the first step in VKOR catalysis of quinone reduction and disulphide-bond generation. Once the Cys133 thiolate is formed, the subsequent reactions become kinetically feasible, as predicted by quantum mechanics calculations of human VKOR [33] . The new structures provide an answer to the physical mechanism of electron transfer in ssVKOR, in which the loop cysteines (Cys50/Cys56) need to move back and forth to reach the two active sites that are 16 Å apart ( Fig. 2 ). How this physical motion can be achieved has been intriguing: Cys56 is attached to exact N -terminal end of the horizontal helix, which forms part of the VKOR active site and is unlikely to move away with Cys56. This apparent mystery can be explained now: the N -terminal part of the horizontal helix can be unwound, which gives Cys56 the flexibility to alternatively interact with Cys50 or Cys130 ( Fig. 3a ). Inserting a few residues between Cys56 and the horizontal helix significantly lowers the efficiency of electron transfer but has little effect on the vitamin K reduction directly at the active site ( Fig. 4 ). In these insertion constructs, it is harder for Cys56 to reach the wound conformation, explaining why the electron transfer is hindered. From these data, we propose a model in which the horizontal helix acts as spring to facilitate electron transfer by undergoing winding and unwinding motions during the redox cycle. These different conformations may be achieved by thermal motions, although the wound conformation is probably more energetically favourable because residues in the horizontal helix form more hydrogen bonds and have more interactions with the membrane at this state. Compared with other disulphide-bond-forming enzymes [13] , [34] , motion of a horizontal helix is a unique feature observed in the VKOR enzyme. Electron transfer in VKOR or DsbB needs to ensure the accessibility of the loop cysteines to their active site buried in a hydrophobic membrane environment. Probably as a result of convergent evolution, both VKOR and DsbB employ a horizontal helix to tether loop cysteines close to the membrane. Compared with DsbB [19] , [35] , the horizontal helix in VKOR is shorter, less buried in the membrane and contains fewer hydrophobic residues ( Supplementary Fig. 4a,b ). In addition, the horizontal helix in DsbB is distant from its active site, whereas in VKOR the horizontal helix forms part of the quinone-binding pocket. The horizontal helix is an immobile anchor in DsbB; however, it is a strikingly dynamic component of VKOR that participates in the process of electron transfer. The unwinding motion of the horizontal helix in VKOR keeps the hydrophobic residues facing the active site and thus only causes a slight disturbance to the local hydrophobic environment. The hydrophobic pocket is thus sealed from solvent access; this is an important mechanism to improve the reactivity of the catalytic cysteine. In human VKOR, the hydrophobic pocket may have the additional function of protecting the highly reactive vitamin K epoxide and hydroquinone. The directionality of the electron transfer in ssVKOR may be partly controlled by the physical separation of Cys50 and Cys56, which are >10 Å apart in the Cys212Ala structure. The Cys50-Cys56 disulphide does not break until it is reduced by the Cys209 in the Trx domain ( Fig. 1a ). The reduction generates a free Cys56 that can be separated from Cys50, which is left behind to form a disulphide with Cys209 (state II). The membrane-association tendency of the horizontal helix probably can drag the Cys56 away from Cys50. This physical separation seems to be an effective way to prevent the backward reaction in which the reduced Cys56 attacks the Cys50-Cys209 disulphide (red arrow in state II). The Cys212Ala structure suggests that the transfer of electrons to the VKOR active site is a one-electron process ( Fig. 6b ). There are two possible outcomes after the free Cys209 reduces the Cys50-Cys56 disulphide: either the reduced Cys56 stays with Cys209-Cys50 until Cys50 is also reduced, or an electron is immediately passed on so that the Cys56 forms a disulphide with Cys130 ( Supplementary Fig. 5 ). The latter state is what has been observed in the Cys212Ala structure, implying that a more stable conformation is to have Cys50 and Cys56 separated. Therefore, electron transfer in ssVKOR may take the following steps: initially, the Cys50-Cys56 disulphide is reduced, generating an intermediate with Cys212 and Cys56 taking the sulfhydryls. The reduced Cys56 is immediately dragged away by the horizontal helix, leaving behind the Cys209-Cys50 disulphide. Next, the free Cys56 interacts with Cys130-Cys133 at the VKOR active site. Importantly, only one electron is transferred during this process, likely resulting in a semi-reduced quinone. To achieve full reduction, the second electron has to be passed on, which starts with the reduction of the Cys209-Cys50 disulphide by the free Cys212. The reduced Cys50 is now free to attack the Cys56-Cys130 disulphide. Therefore, instead of being fully reduced, the loop cysteines transfer one electron at a time through the formation of different disulphides. Functional importance of the flexible horizontal helix suggests a novel explanation for warfarin resistance. Several warfarin-resistant mutations (Asp36Tyr, Val45Ala, Ser52Trp/Leu, Val54Leu, Ser56Phe, Arg58Gly, Trp59Leu/Arg/Cys, Val66Met/Gly, Gly71/Ala and Asn77Tyr/Ser) identified in human and rodent VKORs [20] , [21] , [22] are distributed between TM1 and TM2 ( Fig. 5b ). How these mutations affect VKOR activity has been unclear because they do not map to the active site that likely binds warfarin [20] , [21] , [22] . We found that several of the corresponding warfarin-resistant mutations in ssVKOR alter the membrane accessibility of a buried residue in the horizontal helix ( Fig. 5c ). As the horizontal helix is located at the membrane surface, a conformational change or movement of the helix can be detected by the change in the membrane accessibility of the buried residue. Since the horizontal helix forms part of the active site, this conformational change may weaken warfarin binding. Therefore, there seems to be two distinct mechanisms causing warfarin resistance: mutations around the active site (for example, Tyr139Phe) in human VKOR may directly prohibit warfarin binding, and mutations between TM1 and TM2 (for example, Arg58Gly) may induce a conformational change of the horizontal helix region. Movement of this helix alters the putative warfarin-binding pocket, resulting in warfarin resistance. In summary, the VKOR-catalysed disulphide formation and exchange uses very different mechanisms compared with DsbB. Unlike DsbB, motions of the horizontal helix in VKOR promote and control electron transfer while maintaining the hydrophobic active site important for catalysis. Mutations nearby this flexible horizontal helix may alter the putative binding pocket of warfarin, suggesting an explanation for warfarin resistance. In future studies, it will be interesting to see whether the human VKOR uses the similar mechanisms. Protein purification and crystallization The Cys50Ala and Cys212Ala mutants of the VKOR homologue from Synechococcus sp. were both expressed in a BL21(DE3) Escherichia coli strain. The membrane fraction was solubilized in 1% dodecyl-β-D-maltopyranoside (DDM), 20 mM Tris/HCl pH 7.5, 0.3 M NaCl and 10% glycerol. The detergent soluble fraction was incubated with Ni-affinity resin and eluted in a buffer containing 20 mM Tris/HCl pH 7.5, 0.1 M NaCl, 0.04% DDM and 0.3 M imidazole. The subsequent gel filtration chromatography was in the same buffer without imidazole and the two mutant proteins were concentrated to about 20 mg ml −1 . The Cys50Ala protein was crystallized in 12% PEG3350, 0.1 M sodium cacodylate, pH 5.5. The crystals were grown at 22 °C using a sitting-drop vapour-diffusion method and 25% glycerol was initially used as the cryoprotectant for freezing in liquid nitrogen. We systematically tested the dehydration of these crystals using small molecular-weight PEGs. This was based on our observation that using PEG400 as a cryoprotectant changed the unit cell dimensions of the crystals. After extensive trials, we found that the best result was achieved by a slow dehydration, in which PEG300 was added in 5% steps every 12 h to a final concentration of 40%. The crystals were directly frozen in liquid nitrogen after the PEG300 dehydration. With the use of this protocol, the crystal diffraction improved from 3.6 to 2.8 Å. The Cys212Ala mutant was crystallized in high concentrations of lipid and detergent [17] . A 20-mg ml −1 protein solution was mixed overnight with 15 mg ml −1 1,2-dioleoyl-sn-glycero-3-phosphocholine and 0.5% DDM. This mixture was crystallized at 22 ° C in hanging drop with a buffer containing 11% PEG1500, 8% glycerol, 5% ethanol, 0.1 M MgCl 2 , 0.1 M NaCl and 0.1 M sodium cacodylate, pH 5.5. The crystals were flash-frozen in liquid nitrogen. Structure determination The Cys50Ala crystals initially diffracted to 3.6 Å in a C222 1 space group ( Supplementary Fig. 1a ). Molecular replacement solutions were obtained by the Phaser program [36] , which searched for the VKOR domain (residues 1–173) and Trx domain (residues 188–283) from the Cys56Ala structure model [14] . The C222 1 crystals contained one molecule of the VKOR-Trx in the asymmetric unit. Omit maps were subsequently calculated using Refmac [37] by rigid body refinement of partial models, in which transmembrane helices and loops were systematically deleted. The omit maps were sharpened by a B factor of −80 Å 2 , and solvent flattening of the maps was calculated by the Parrot program [38] . An omit map with the deletion of residues 43–73 regenerated electron densities that suggested a different conformation of the loop/helix region connecting TM1 and TM2. The structural model was built manually in Coot [39] and refined by the Refmac program using data corrected for anisotropy. Dehydration of the crystals improved the diffraction to 2.8 Å ( Supplementary Fig. 1a ) and changed the space group to C2 ( Supplementary Fig. 1b ). One of the unit cell dimensions shrunk from 131 to 119 Å. Molecular replacement found two molecules in the asymmetric unit, which resulted from the breakdown of a twofold crystal symmetry in the C222 1 crystals ( Supplementary Fig. 1b ). A series of omit maps with deletions mentioned above were calculated, and an initial model was built from these maps. The maps calculated from the C2 data were very similar to that from the C222 1 data, except that side chain densities were better defined in the 2.8-Å map ( Fig. 3b ) and residues 49–53 in the electron-transfer loop could not be built from this map. However, restrained refinement of these models resulted in R factors >40%. Refinement using a Detwin process installed in Refmac significantly lowered the R factors, and the twinning fraction was refined to 36%. The detwinned data were sharpened by a B factor of −30 Å 2 , and the omit maps were averaged using the twofold noncrystallographic symmetry by the Parrot program. The averaged omit maps were used to build a 2.8-Å model, which was refined against the detwinned data to R and R free of 23.2% and 24.5%, respectively. At this stage, composite omit maps were calculated using a torsion-angle-simulated annealing method installed in the CNS program suite [40] . The refined model fits well with the composite omit maps. The crystals of Cys212Ala mutant diffracted to 4.2 Å in a P6 1 space group. The VKOR and Trx domains from the 2.8-Å Cys50Ala model were used for MR and for generating omit maps. The omit maps were improved by solvent flattening (80% solvent content) using the Parrot program. Electron density for the entire loop/helix region was regenerated ( Supplementary Fig. 2 ), which had been deleted in the model. Owing to its higher accuracy, the 2.8-Å model was also used to re-calculate model maps for the 3.6-Å Cys56Ala data. We first confirmed the conformation of the loop/helix region by Fo-Fc and 2Fo-Fc maps, which were generated after rigid body refinement by Refmac. The Fo-Fc map contoured at 3 sigma shows the positive densities of the electron-transfer loop in its real conformation and negative densities of the wrong positions in the MR model. We also calculated omit maps by deleting the region (residues 44–77) of the electron-transfer loop and horizontal helix. After solvent-flattening, the omit maps ( Supplementary Fig. 6 ) were very similar to maps obtained previously by experimental phasing methods using a 3.6-Å data set of a mercury derivative [14] . Thus, these independent phasing methods generated very similar maps, confirming the conformation changes of the horizontal helix and the electron-transfer loop. Activity assay Reduction of vitamin K was measured using a fluorometric assay [14] with the following modifications. The VKOR protein was first incubated with 5 mM DTT (or 0.05 mM of reduced and unfolded RNaseA) to completely reduce the endogenous quinone, and 0.2 mM vitamin K was subsequently added to initiate the reaction. To avoid filtering effect from the protein, the excitation and emission wavelength were changed to 330 nm and 430 nm, respectively. Probing of membrane accessibility Membrane accessibility of residues on the horizontal helix ( Supplementary Fig. 7 ) was detected by an established protocol [18] , [19] . The warfarin-resistant mutation was generated on a truncated ssVKOR construct (residues 1–182) with multiple mutations of Leu60Cys, Cys50Ala, Cys56Ala, Cys130Ala and Cys133Ala. In other words, only the VKOR domain is used and all endogenous cysteines have been mutated to alanine. Cells overexpressing the mutant proteins were lysed by lysozyme to generate sphereoplast. A membrane-impermeable probe, AMS, was used to label exposed cysteines. Subsequently, the proteins were denatured by TCA precipitation, and MalPEG (5 KDa) was used to label unblocked cysteines from the previous step. How to cite this article: Liu, S. et al . Structures of an intramembrane vitamin K epoxide reductase homologue reveal control mechanisms for electron transfer. Nat. Commun. 5:3110 doi: 10.1038/ncomms4110 (2014). Accession codes : The structure factors and coordinates have been deposited in the protein data bank (accession codes 4NV5 and 4NV2 for the Cys50Ala structure and accession code 4NV6 for the Cys212Ala structure).